Parkin controls dopamine utilization in human midbrain dopaminergic neurons derived from induced pluripotent stem cells Parkinson's disease (PD) is defined by the degeneration of nigral dopaminergic (DA) neurons and can be caused by monogenic mutations of genes such as parkin. The lack of phenotype in parkin knockout mice suggests that human nigral DA neurons have unique vulnerabilities. Here we generate induced pluripotent stem cells from normal subjects and PD patients with parkin mutations. We demonstrate that loss of parkin in human midbrain DA neurons greatly increases the transcription of monoamine oxidases and oxidative stress, significantly reduces DA uptake and increases spontaneous DA release. Lentiviral expression of parkin, but not its PD-linked mutant, rescues these phenotypes. The results suggest that parkin controls dopamine utilization in human midbrain DA neurons by enhancing the precision of DA neurotransmission and suppressing dopamine oxidation. Thus, the study provides novel targets and a physiologically relevant screening platform for disease-modifying therapies of PD. Parkinson's disease (PD) is clinically defined by a core set of motor symptoms that are believed to be caused by the degeneration of dopaminergic (DA) neurons in substantia nigra [1] . A variety of environmental and genetic factors underlie the accelerated degeneration of nigral DA neurons in PD [2] . Although monogenic forms of PD account for a small percentage of cases [2] , understanding how mutations of these genes lead to the selective degeneration of nigral DA neurons holds great promise to the discovery of disease-modifying therapies for PD. Among the genes that have been causatively linked to PD, parkin is unique in that its mutations are most frequently found in recessively inherited PD cases; they are completely penetrant and do not have a founder effect [3] . Parkin is an ubiquitin-protein ligase [4] for a variety of substrates [5] . In sharp contrast to the situation seen in PD patients with parkin mutations [6] , parkin knockout mice do not exhibit any robust phenotype [7] , suggesting that parkin mutations selectively impact on human nigral DA neurons. One of the major roadblocks in PD research is the lack of live human midbrain DA neurons. The discovery of human induced pluripotent stem cells (iPSCs) [8] , [9] has allowed us in this study to generate patient-specific iPSCs, which were differentiated in vitro to midbrain DA neurons for mechanistic studies of parkin. We find that parkin mutations in iPSC-derived human midbrain DA neurons significantly elevates oxidative stress induced by dopamine oxidation because the transcription of monoamine oxidases A and B greatly increases. Specific dopamine uptake through dopamine transporter (DAT) significantly decreases, as the amounts of DAT-binding sites significantly reduce. In addition, spontaneous Ca 2+ -independent release of dopamine significantly increases while activity- and Ca 2+ -dependent DA release remains the same. These dopamine-specific phenotypes can be significantly reversed by lentiviral expression of wild-type parkin, but not its PD-linked T240R mutant or green fluorescent protein (GFP). The results not only reveal mechanistic insights into the cellular functions of parkin in human midbrain DA neurons—the cell type selectively impacted by its mutations, they also provide novel targets and a screening platform for the discovery of disease-modifying agents that can mimic the protective functions of parkin. Generation of iPSCs from PD patients with parkin mutations To understand why mutations of parkin cause the selective degeneration of human nigral DA neurons and ensuing PD [6] , we generated iPSCs using dermal fibroblasts from two PD patients with parkin mutations (one with compound heterozygous deletions of exon 3 and exon 5, designated as P001; the other with homozygous deletion of exon 3, designated as P002) and two control subjects (designated as C001 and C002) who are unrelated, unaffected spouses of idiopathic PD patients. Dermal fibroblasts cultured from skin punch biopsy were reprogrammed to iPSCs using lentiviruses expressing human Oct4, Sox2, Klf4, c-Myc and Nanog [10] . Multiple clones with human embryonic stem cell (hESC) morphology were picked for each of the four subjects. After expansion and initial characterization, one representative clone for each subject (C001#2, C002#1, P001#3, P002#4.5) was used for detailed studies. 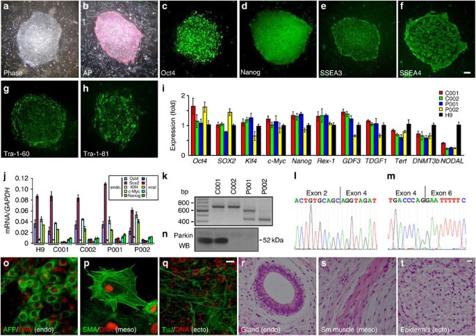Figure 1: Generation of induced pluripotent stem cells (iPSCs) from normal subjects and PD patients with parkin mutations. (a–h) Phase contrast image (a) of P002 iPSCs from a PD patient with parkin mutations and staining of the line with pluripotency markers alkaline phosphatase (AP) (b), Oct4 (c), Nanog (d), SSEA3 (e), SSEA4 (f), Tra-1-60 (g) and Tra-1-81 (h). Bar, 100 μm. (i) Expression levels of endogenous pluripotency genes in the four representative iPSC lines and H9 human embryonic stem cell (hESC). (j) Levels of viral transgenes and their endogenous counterparts in the four iPSC lines and H9 hESC. Error bars in (i) and (j) represent s.e.m.,n=9. (k–m) Real-time PCR amplification of the parkin transcripts in the four iPSC lines (k) and sequencing results of the band with exon 3 deletion (l) and the band with exon 5 deletion (m). (n) Parkin immunoblot of total cell lysates from the four lines of iPSCs. (o–q) EB-mediated spontaneous differentiation of P002 iPSCsin vitro. Bar, 10 μm. (r–t) Teratoma formation assay for P002 iPSCs. ecto, ectoderm; endo, endoderm; meso, mesoderm; Sm, smooth. Bar, 10 μm. As shown in Figure 1 for P002 iPSC and Supplementary Figure S1 for the other three lines, all four lines of iPSCs exhibited morphology indistinguishable from hESCs such as H9 and can be maintained indefinitely on mouse embryonic fibroblast feeders or matrigel. Pluripotency markers such as alkaline phosphatase, Oct4, Nanog, SSEA3, SSEA4, Tra-1-60 and Tra-1-81 were strongly expressed in all four lines. Real-time quantitative reverse transcriptase PCR (qRT–PCR) showed that a panel of endogenous pluripotency genes (except NODAL ) were expressed at levels comparable to those in H9 hESC ( Fig. 1i and Supplementary Fig. S1y ). Sequences of PCR primers are listed in Supplementary Table S1 . The reason for the low level of NODAL is unclear and might be related to our iPSC-derivation method and condition (for example, we used 5% O 2 in iPSC derivation and culture). DNA methylation in the promoter regions of Oct4, Nanog and Sox2 was greatly reduced in the four lines of iPSCs, in comparison to that in the original fibroblast lines ( Supplementary Fig. S2 ). The promoter sequences are listed in Supplementary Table S2 . The five viral transgenes were strongly silenced in these iPSCs ( Fig. 1j ; Supplementary Fig. S1y ). RT–PCR was performed on total RNA from the four lines of iPSCs grown on matrigel to confirm parkin mutations in the two PD patients ( Fig. 1k ). The RT–PCR products were sequenced to verify that P001 iPSC indeed had compound heterozygous deletions of exon 3 and exon 5 while P002 iPSC had homozygous deletion of exon 3 ( Fig. 1l,m ). Western blotting of total cell lysates from the four lines of iPSCs confirmed that parkin was not expressed in P001 and P002 cells ( Fig. 1n ). In embryoid body-mediated spontaneous differentiation assays, all four lines of iPSCs could be differentiated to cells of the three germ layers ( Fig. 1o–q for P002 and Supplementary Fig. S3 for the other three lines). They also formed teratomas under kidney capsules in SCID mice ( Fig. 1r–t for P002 and Supplementary Fig. S3 for the other three lines). All four lines of iPSCs showed normal karyotypes ( Supplementary Fig. S4 ). This was confirmed by array comparative genomic hybridization, which showed no significant chromosomal change in the iPSCs when compared with pooled normal human genomic DNA ( Supplementary Fig. S5 ). Figure 1: Generation of induced pluripotent stem cells (iPSCs) from normal subjects and PD patients with parkin mutations. ( a – h ) Phase contrast image ( a ) of P002 iPSCs from a PD patient with parkin mutations and staining of the line with pluripotency markers alkaline phosphatase (AP) ( b ), Oct4 ( c ), Nanog ( d ), SSEA3 ( e ), SSEA4 ( f ), Tra-1-60 ( g ) and Tra-1-81 ( h ). Bar, 100 μm. ( i ) Expression levels of endogenous pluripotency genes in the four representative iPSC lines and H9 human embryonic stem cell (hESC). ( j ) Levels of viral transgenes and their endogenous counterparts in the four iPSC lines and H9 hESC. Error bars in ( i ) and ( j ) represent s.e.m., n =9. ( k–m ) Real-time PCR amplification of the parkin transcripts in the four iPSC lines ( k ) and sequencing results of the band with exon 3 deletion ( l ) and the band with exon 5 deletion ( m ). ( n ) Parkin immunoblot of total cell lysates from the four lines of iPSCs. ( o–q ) EB-mediated spontaneous differentiation of P002 iPSCs in vitro . Bar, 10 μm. ( r–t ) Teratoma formation assay for P002 iPSCs. ecto, ectoderm; endo, endoderm; meso, mesoderm; Sm, smooth. Bar, 10 μm. Full size image Differentiation of iPSCs to midbrain DA neurons We used a feeder-free, chemically defined, directed differentiation protocol [11] to differentiate the four lines of iPSCs to midbrain DA neurons in vitro ( Fig. 2 ). The iPSC colonies dissociated from mouse embryonic fibroblast cells were first cultured as floating cell aggregates (EB) for 4 days in hESC medium with 10 μM SB431542 to enhance neural differentiation [12] . After the cell aggregates were cultured in suspension in the presence of 20 ng ml −1 bFGF for two more days, they were plated on laminin-coated surface. Many colonies had an elongated columnar morphology. These primitive neuroepithelial cells were differentiated to definitive neuroepithelia in the presence of FGF8a (20 ng ml −1 ) and SHH (100 ng ml −1 ). Multiple neural tube-like rosettes were seen in the centre of the colony ( Fig. 2b ). The rosettes were peeled off from the flat peripheral cells and cultured in suspension in the presence of FGF8a (50 ng ml −1 ) and SHH (100 ng ml −1 ), B27 supplements (1×) and ascorbic acid (200 μM) to form neurospheres that were patterned to a mid/hind brain destiny ( Fig. 2c ). Around day 24, the neurospheres were dissociated and plated on 6-well plates or cover slips precoated with polyornithine, laminin and matrigel. We found that the addition of matrigel coating significantly inhibited the formation of cell aggregates during the last step of differentiation and might have contributed to the improved DA characteristics, such as specific dopamine uptake. Trophic factors such as BDNF (20 ng ml −1 ) and GDNF (20 ng ml −1 ) were used to generate mature DA neurons, which were seen around 70 days from the start of differentiation ( Fig. 2d ). 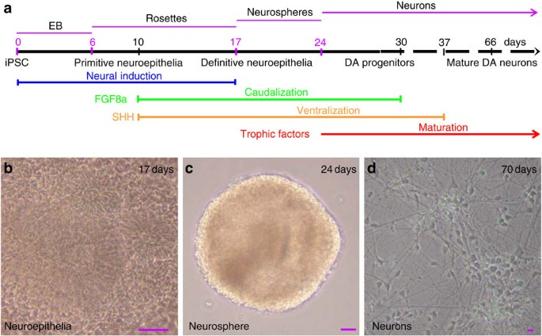Figure 2: Directed differentiation of the induced pluripotent stem cells (iPSCs) to midbrain dopaminergic (DA) neuronsin vitro. (a–d) iPSCs were differentiated with the protocol in (a) to neuroepithelia (b), neurosphere (c) and neurons (d). Bars, 100 μm in (b) and (c), and 10 μm in (d). Figure 2: Directed differentiation of the induced pluripotent stem cells (iPSCs) to midbrain dopaminergic (DA) neurons in vitro . ( a–d ) iPSCs were differentiated with the protocol in ( a ) to neuroepithelia ( b ), neurosphere ( c ) and neurons ( d ). Bars, 100 μm in ( b ) and ( c ), and 10 μm in ( d ). Full size image P002 iPSC-derived neuronal cultures contained TH + neurons with complex morphology and in clusters (for example, Fig. 3a,b ). These TH + neurons expressed the midbrain markers engrailed-1 (En-1) [13] ( Fig. 3a ) and FoxA2 ( Fig. 3b ), as well as other DA markers such as AADC ( Fig. 3c ), DAT ( Fig. 3d ) and VMAT2 ( Fig. 3e ), suggesting that they are midbrain DA neurons. They expressed synaptic markers such as synaptophysin ( Fig. 3f ) and NR1 ( Fig. 3g ), and markers for mature neurons such as MAP2 ( Fig. 3h ). Similar expression of these markers was seen in neuronal cultures derived from C001, C002 and P001 iPSC lines ( Supplementary Fig. S6 ). Consistent with this, RT–PCR experiments showed that TH, En-1, AADC, DAT, VMAT2, Nurr1, Ptx3, FoxA2 and Lmx1b were strongly expressed in iPSC-derived neurons, but not in the iPSCs ( Supplementary Fig. S7 ). The weak expression of FoxA2 and Lmx1b in our iPSCs was similar to what has been reported before [14] , [15] . qRT–PCR experiments showed that there were very low levels of viral transgene expression in the four lines of iPSC-derived neurons ( Supplementary Fig. S8 ). Similar to what has been reported recently for the differentiation of iPSCs to motor neurons [16] , the low level of transgene expression in our iPSC-derived neurons did not appear to affect the differentiation or function of these neurons, as electrophysiological studies showed that P002 neurons fired spontaneous action potentials (APs; Fig. 3i ) and evoked APs ( Fig. 3j ). They have voltage-gated K + currents and voltage-gated Na + currents ( Fig. 3k ), N -methyl- D -aspartic acid (NMDA)-gated currents ( Fig. 3l ), γ-aminobutyric acid (GABA)-gated currents ( Fig. 3m ) and spontaneous excitatory postsynaptic currents ( Fig. 3n ). Similar electrophysiological profiles were observed in neurons derived from C001, C002 and P001 iPSCs ( Supplementary Fig. S9 ). These results showed that all four lines of iPSC-derived neuronal cultures had synaptic transmission and contained midbrain DA neurons. 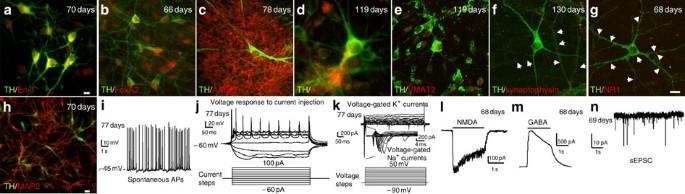Figure 3: Properties of the induced pluripotent stem cell (iPSC)-derived midbrain dopaminergic (DA) neurons. (a–h) P002 iPSC-derived neuronal cultures were co-stained for TH and the midbrain markers engrailed-1 (En-1) (a) and FoxA2 (b), the DA markers AADC (c), dopamine transporter (DAT) (d) and VMAT2 (e), the synaptic markers synaptophysin (f) and NR1 (g), and the marker for mature neurons MAP2 (h). Bars, 10 μm. (i–n) These neurons fired spontaneous APs (i) and evoked APs (j), had voltage-gated K+and Na+currents (k),N-methyl-D-aspartic acid (NMDA)-gated currents (l), γ-aminobutyric acid (GABA)-gated currents (m) and spontaneous EPSC (n). Dates (for example, 70 days) indicated were from the start of differentiation. AP, action potential; sEPSC, spontaneous excitatory postsynaptic currents. Figure 3: Properties of the induced pluripotent stem cell (iPSC)-derived midbrain dopaminergic (DA) neurons. ( a – h ) P002 iPSC-derived neuronal cultures were co-stained for TH and the midbrain markers engrailed-1 (En-1) ( a ) and FoxA2 ( b ), the DA markers AADC ( c ), dopamine transporter (DAT) ( d ) and VMAT2 ( e ), the synaptic markers synaptophysin ( f ) and NR1 ( g ), and the marker for mature neurons MAP2 ( h ). Bars, 10 μm. ( i–n ) These neurons fired spontaneous APs ( i ) and evoked APs ( j ), had voltage-gated K + and Na + currents ( k ), N -methyl- D -aspartic acid (NMDA)-gated currents ( l ), γ-aminobutyric acid (GABA)-gated currents ( m ) and spontaneous EPSC ( n ). Dates (for example, 70 days) indicated were from the start of differentiation. AP, action potential; sEPSC, spontaneous excitatory postsynaptic currents. Full size image Parkin mutations increased spontaneous DA release To demonstrate that these midbrain DA neurons are functional, we measured spontaneous and activity-dependent dopamine release by reverse phase high pressure liquid chromatography (HPLC) coupled with electrochemical detection of dopamine [17] . The iPSC-derived neuronal cultures were incubated at 37°C in Hank's Balanced Salt Solution (HBSS), HBSS with 56 mM KCl or Ca 2+ -free HBSS with 56 mM KCl. Spontaneous DA release in HBSS (30 min) was robustly observed in all four lines of iPSC-derived DA neurons and was significantly increased in P001 and P002, compared with C001 or C002 ( P <0.05, n =3–8, Student's t -test, unpaired, two-tailed) ( Fig. 4a ). DA release was markedly increased by KCl-induced membrane depolarization in the four lines of DA neurons, and the increases were abolished when Ca 2+ -free HBSS was used with KCl ( Fig. 4a ). Ca 2+ - and activity-dependent release was calculated by the difference between KCl-induced DA release in the presence and absence of Ca 2+ ; it was not significantly different among the four lines of DA neurons ( Fig. 4b ). To ascertain that increased spontaneous DA release was indeed caused by the loss of parkin, we infected P001 or P002 neurons with lentivirus expressing GFP or FLAG-tagged parkin or its PD-linked T240R mutant. Overexpression of wild-type parkin, but not its T240R mutant or GFP, significantly reduced spontaneous DA release in HBSS from P001 or P002 neurons ( P <0.05 versus P001 or P002 expressing GFP, respectively, n =4, Student's t -test, unpaired, two-tailed) ( Fig. 4c ). The spontaneous dopamine release was not significantly affected by selective inhibitors of DAT such as GBR12909 (10 μM) or nomifensine (10 μM) ( Supplementary Fig. S10a ), suggesting that it is not caused by dopamine efflux through DAT. Total dopamine content in these neuronal cultures as measured by HPLC was not significantly different ( Fig. 4d ). We counted more than 1000 NeuN + neurons for each line. The percentage of TH + neurons in NeuN + neurons was not significantly different ( Fig. 4e ). We plated the same number of neuroepithelial cells at the last step of differentiation. The total number of neurons were too numerous to count. Thus, the similar percentages of TH + neurons suggest that the numbers of DA neurons are similar across the four lines. 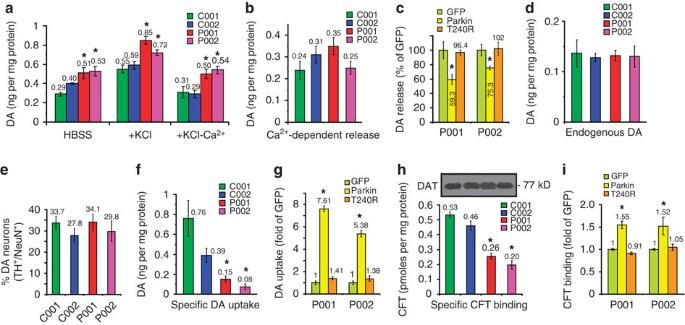Figure 4: Dopamine release and uptake in the four lines of induced pluripotent stem cell (iPSC)-derived midbrain dopaminergic (DA) neurons. (a) Dopamine release in Hank's Balanced Salt Solution (HBSS), or in HBSS plus KCl (56 mM), or Ca2+-free HBSS plus KCl (56 mM) from normal and parkin-deficient iPSC-derived midbrain neuronal cultures. *P<0.05 versus C001 or C002 in the same condition,n=3–8, Student'st-test, unpaired, two-tailed. (b) Ca2+-dependent DA release was calculated from KCl-induced DA release in the presence or absence of Ca2+. (c) Spontaneous DA release in HBSS from P001 or P002 neurons infected with lentivirus expressing green fluorescent protein (GFP), parkin or T240R mutant parkin. *P<0.05 versus P001 or P002 expressing GFP, respectively,n=4, Student'st-test, unpaired, two-tailed. (d,e) The amount of endogenous dopamine (d) and the percentage of TH+neurons in NeuN+neurons (e) in the four lines of iPSC-derived neuronal cultures. At least 1000 NeuN+neurons were counted for each line of the iPSC-derived neurons. (f) Specific dopamine uptake in the four lines of iPSC-derived midbrain neuronal cultures. *P<0.05 versus C001 or C002,n=5–9, Student'st-test, unpaired, two-tailed. (g) Specific DA uptake in P001 or P002 neurons infected with lentivirus expressing GFP, parkin or T240R mutant parkin. *P<0.05 versus P001 or P002 expressing GFP, respectively,n=4, Student'st-test, unpaired, two-tailed. (h) Specific [3H]CFT binding on dopamine transporter (DAT) in the four lines of iPSC-derived midbrain neuronal cultures. *P<0.05 versus C001 or C002,n=6, Student'st-test, unpaired, two-tailed. (i) Specific [3H]CFT binding in P001 or P002 neurons infected with lentivirus expressing GFP, parkin or T240R mutant parkin. *P<0.05 versus P001 or P002 expressing GFP, respectively,n=5, Student'st-test, unpaired, two-tailed. Error bars represent s.e.m. Figure 4: Dopamine release and uptake in the four lines of induced pluripotent stem cell (iPSC)-derived midbrain dopaminergic (DA) neurons. ( a ) Dopamine release in Hank's Balanced Salt Solution (HBSS), or in HBSS plus KCl (56 mM), or Ca 2+ -free HBSS plus KCl (56 mM) from normal and parkin-deficient iPSC-derived midbrain neuronal cultures. * P <0.05 versus C001 or C002 in the same condition, n =3–8, Student's t -test, unpaired, two-tailed. ( b ) Ca 2+ -dependent DA release was calculated from KCl-induced DA release in the presence or absence of Ca 2+ . ( c ) Spontaneous DA release in HBSS from P001 or P002 neurons infected with lentivirus expressing green fluorescent protein (GFP), parkin or T240R mutant parkin. * P <0.05 versus P001 or P002 expressing GFP, respectively, n =4, Student's t -test, unpaired, two-tailed. ( d,e ) The amount of endogenous dopamine ( d ) and the percentage of TH + neurons in NeuN + neurons ( e ) in the four lines of iPSC-derived neuronal cultures. At least 1000 NeuN + neurons were counted for each line of the iPSC-derived neurons. ( f ) Specific dopamine uptake in the four lines of iPSC-derived midbrain neuronal cultures. * P <0.05 versus C001 or C002, n =5–9, Student's t -test, unpaired, two-tailed. ( g ) Specific DA uptake in P001 or P002 neurons infected with lentivirus expressing GFP, parkin or T240R mutant parkin. * P <0.05 versus P001 or P002 expressing GFP, respectively, n =4, Student's t -test, unpaired, two-tailed. ( h ) Specific [ 3 H]CFT binding on dopamine transporter (DAT) in the four lines of iPSC-derived midbrain neuronal cultures. * P <0.05 versus C001 or C002, n =6, Student's t -test, unpaired, two-tailed. ( i ) Specific [ 3 H]CFT binding in P001 or P002 neurons infected with lentivirus expressing GFP, parkin or T240R mutant parkin. * P <0.05 versus P001 or P002 expressing GFP, respectively, n =5, Student's t -test, unpaired, two-tailed. Error bars represent s.e.m. Full size image Parkin mutations decreased DA uptake and DAT-binding sites We measured specific DA uptake by incubating the neuronal cultures for 10 min at 37°C with 5 μM dopamine in the absence or presence of 10 μM nomifensine, a selective inhibitor of DAT. The condition was based on the dose response and time course of dopamine uptake in C001 neurons ( Supplementary Fig. S10b,c ). The ligand concentration (5 μM) was very close to V max condition and the duration (10 min) was in the linear phase of uptake. It was used before in our previous study [18] and was consistent with other studies using cloned human DAT in exogenous expression systems [19] , [20] . The amount of dopamine in the cells as measured by HPLC was used to calculate specific DA uptake, which is the difference of DA uptake in the absence and presence of nomifensine. Non-specific DA uptake in the presence of nomifensine was not significantly different between the four lines of iPSC-derived neurons (data not shown). Furthermore, dopamine uptake was not significantly affected by nisoxetine (0.1 μM), a selective inhibitor of norepinephrine transporter ( Supplementary Fig. S10d ). As shown in Figure 4f , specific DA uptake was significantly diminished in P001 and P002 DA neurons, compared with C001 or C002 DA neurons ( P <0.05, n =5–9, Student's t -test, unpaired, two-tailed). Lentiviral expression of parkin, but not its T240R mutant or GFP, significantly rescued the effect ( P <0.05 versus P001 or P002 expressing GFP, respectively, n =4, Student's t -test, unpaired, two-tailed) ( Fig. 4g ), suggesting that the effect is indeed caused by loss-of-function mutations of parkin in P001 and P002 neurons. Our previous study has shown that parkin enhances the cell surface expression of DAT by ubiquitinating and degrading misfolded DAT to facilitate the oligomerization of native DAT conformers in the endoplasmic reticulum [18] , a prerequisite for the plasma membrane delivery of this misfolding-prone protein [21] . To test whether reduced dopamine uptake in P001 and P002 neurons is caused by a decreased amount of correctly folded DAT that are competent for selective dopamine uptake, we measured the amounts of DAT-binding sites using [ 3 H]CFT [2-β-carbomethoxy-3-beta-(4-fluorophenyl)-tropane] [18] , a potent cocaine analogue that specifically binds to DAT. The iPSC-derived neuronal cultures were incubated for 2 h at 4°C in binding buffer with 4 nM [ 3 H]CFT in the absence or presence of the selective DAT inhibitor GBR12909 (10 μM). Total cell lysates, in which [ 3 H]CFT was bound to correctly folded DAT molecules, were measured in a scintillation counter to calculate specific [ 3 H]CFT binding on DAT (the difference in binding with or without GBR12909). As shown in Figure 4h , specific [ 3 H]CFT binding was greatly reduced in P001 and P002 DA neurons, compared with C001 or C002 DA neurons ( P <0.05, n =6, Student's t -test, unpaired, two-tailed), while the levels of total DAT in whole-cell lysates were very similar. To confirm that reduced DAT-binding sites were indeed caused by parkin mutations in P001 and P002 neurons, we infected these neurons with lentivirus expressing GFP, parkin or its PD-linked T240R mutant. As shown in Figure 4i , overexpression of parkin, but not T240R or GFP, significantly increased the specific binding of [ 3 H]CFT in P001 or P002 neurons ( P <0.05 versus P001 or P002 expressing GFP, respectively, n =5, Student's t -test, unpaired, two-tailed). Parkin mutations elevated ROS by increasing MAO transcripts To test the impact of parkin mutations on dopamine-induced oxidative stress, which has a key role in the selective degeneration of nigral DA neurons in PD [22] , we treated the four lines of iPSC-derived neuronal cultures without or with 75 μM dopamine for 4 h, and examined the level of oxidative stress by measuring the amounts of protein carbonyls in the total cell lysates. Without dopamine treatment, very few protein carbonyls were seen in all four lines of human neurons. After DA treatment, the amounts of protein carbonyls were greatly increased in P001 and P002 neurons, compared with those in C001 or C002 neurons ( P <0.01, n =8, Student's t -test, unpaired, two-tailed), which only had very modest increases over their basal levels ( Fig. 5a,b ). The results suggest that dopamine-induced oxidative stress is markedly elevated when parkin is mutated. Our previous study has shown that parkin suppresses the transcription of monoamine oxidases (MAO) A and B [17] , which are mitochondrial enzymes responsible for the oxidative deamination of dopamine, a reaction that produces large quantities of reactive oxygen species [23] . When we measured the messenger RNA levels of MAO-A and MAO-B by qRT–PCR, we found that the amounts of MAO-A and MAO-B transcripts were significantly increased in P001 and P002 neurons, compared with those in C001 or C002 neurons ( P <0.01, n =9, Student's t -test, unpaired, two-tailed) ( Fig. 5c ). To substantiate these findings, we measured the activities of MAO-A or MAO-B in total cell lysates from these neurons using [ 14 C]tyramine as a substrate, and pargyline or clorgyline to inhibit MAO-B or MAO-A, respectively [17] . 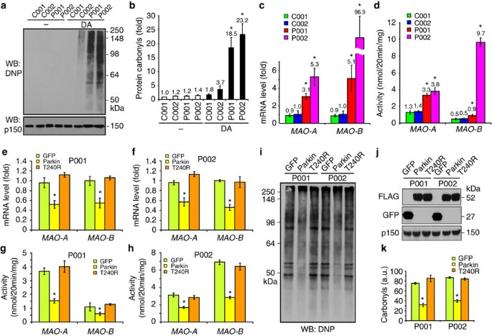Figure 5: Oxidative stress and monoamine oxidase (MAO) transcription in the four lines of induced pluripotent stem cell (iPSC)-derived neurons. (a,b) Western blot analysis (a) and quantification (b) of protein carbonyls in the four lines of iPSC-derived neurons treated without or with dopamine (75 μM for 4 h). DNP, 2,4-dinitrophenyl; p150, p150glued, a dynactin subunit as loading control. *P<0.01 versus C001 or C002 with DA treatment,n=8, Student'st-test, unpaired, two-tailed. (c) Quantitative reverse transcriptase PCR (qRT–PCR) measurement ofMAO-AandMAO-Btranscripts in the four lines of iPSC-derived neuronal cultures. *P<0.01 versus C001 or C002,n=9, Student'st-test, unpaired, two-tailed. (d) MAO-A and MAO-B activities in the four lines of iPSC-derived neurons. *P<0.01 versus C001 or C002,n=6–11, Student'st-test, unpaired, two-tailed. (e,f) qRT–PCR measurements of MAO-A and MAO-B messenger RNA (mRNA) levels in P001 (e) or P002 (f) neurons infected with lentivirus expressing green fluorescent protein (GFP), parkin or T240R mutant parkin. (g,h) MAO-A and MAO-B activities in P001 (g) or P002 (h) neurons infected with lentivirus expressing GFP, parkin or T240R mutant parkin. (i–k) Western blot analysis (i) and quantification (k) of protein carbonyls in P001 or P002 neurons infected with lentivirus expressing GFP, parkin or T240R mutant parkin. Total cell lysates were blotted with antibodies against GFP or FLAG or p150glued(j). *P<0.05 versus GFP-expressing neurons,n=3–4 for (e) to (k), Student'st-test, unpaired, two-tailed. mg, milligrams of total cellular proteins. Error bars represent s.e.m. As shown in Figure 5d , the amounts of MAO-A or MAO-B enzymatic activities were significantly increased in P001 and P002 neurons, compared with those in C001 or C002 neurons ( P <0.01, n =6–11, Student's t -test, unpaired, two-tailed). Figure 5: Oxidative stress and monoamine oxidase (MAO) transcription in the four lines of induced pluripotent stem cell (iPSC)-derived neurons. ( a,b ) Western blot analysis ( a ) and quantification ( b ) of protein carbonyls in the four lines of iPSC-derived neurons treated without or with dopamine (75 μM for 4 h). DNP, 2,4-dinitrophenyl; p150, p150 glued , a dynactin subunit as loading control. * P <0.01 versus C001 or C002 with DA treatment, n =8, Student's t -test, unpaired, two-tailed. ( c ) Quantitative reverse transcriptase PCR (qRT–PCR) measurement of MAO-A and MAO-B transcripts in the four lines of iPSC-derived neuronal cultures. * P <0.01 versus C001 or C002, n =9, Student's t -test, unpaired, two-tailed. ( d ) MAO-A and MAO-B activities in the four lines of iPSC-derived neurons. * P <0.01 versus C001 or C002, n =6–11, Student's t -test, unpaired, two-tailed. ( e,f ) qRT–PCR measurements of MAO-A and MAO-B messenger RNA (mRNA) levels in P001 ( e ) or P002 ( f ) neurons infected with lentivirus expressing green fluorescent protein (GFP), parkin or T240R mutant parkin. ( g,h ) MAO-A and MAO-B activities in P001 ( g ) or P002 ( h ) neurons infected with lentivirus expressing GFP, parkin or T240R mutant parkin. ( i–k ) Western blot analysis ( i ) and quantification ( k ) of protein carbonyls in P001 or P002 neurons infected with lentivirus expressing GFP, parkin or T240R mutant parkin. Total cell lysates were blotted with antibodies against GFP or FLAG or p150 glued ( j ). * P <0.05 versus GFP-expressing neurons, n =3–4 for ( e ) to ( k ), Student's t -test, unpaired, two-tailed. mg, milligrams of total cellular proteins. Error bars represent s.e.m. Full size image To ascertain that these phenotypes were indeed caused by parkin mutations, we infected P001 or P002 neurons with lentivirus expressing GFP, FLAG-tagged parkin or T240R mutant parkin. Overexpression of parkin, but not its PD-linked T240R mutant or GFP, significantly lowered the messenger RNA levels of MAO-A and MAO-B in P001 and P002 neurons ( P <0.05, n =4, Student's t -test, unpaired, two-tailed) ( Fig. 5e,f ), as well as the activities of MAO-A and MAO-B in total cell lysates from these neurons ( P <0.05, n =4, Student's t -test, unpaired, two-tailed) ( Fig. 5g,h ). Consistent with these findings, the amounts of protein carbonyls in P001 and P002 neurons were significantly decreased by overexpression of parkin, but not its T240R mutant or GFP ( P <0.05, n =3, Student's t -test, unpaired, two-tailed) ( Fig. 5i,k ). The expression levels of GFP, FLAG-tagged parkin or its T240R mutant, and p150 glued (as loading control) were shown in Figure 5j . Parkin mutations did not significantly affect mitochondria We examined whether the loss of parkin significantly affect mitochondria by treating the four lines of iPSC-derived neurons without or with CCCP (10 μM for 16 h) to induce mitophagy [24] . There was no significant change in the amount of mitochondria as reflected in the quantitative PCR measurement of mitochondrial DNA against the nuclear gene actin ( Fig. 6a–c ). The protein expression levels of PINK1 and DJ-1 in the presence or absence of CCCP (10 μM for 24 h) were not significantly changed ( Fig. 6d ). The expression levels of α-synuclein were also very similar among the four lines of iPSC-derived neurons ( Fig. 6e ). 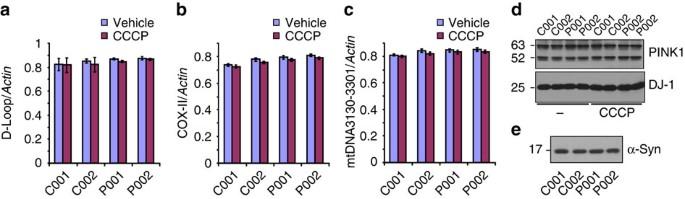Figure 6: Mitochondrial DNA levels and protein expression in the four lines of induced pluripotent stem cell (iPSC)-derived neurons. (a–c) Quantitative PCR measurement of three different segments of mitochondria DNA against the nuclear gene actin in the four lines of iPSC-derived neurons treated with or without CCCP (10 μM for 16 h). mtDNA3130-3301 is a region not transcribed and has no homology with mitochondrial pseudogenes in the nuclear genome. (d) Protein expression levels of PINK1 and DJ-1 in the absence or presence of CCCP treatment (10 μM for 24 h). PINK1 has two bands, uncleaved at 63 kDa and cleaved at 52 KDa. (e) The expression level of α-synuclein in the four lines of iPSC-derived neurons. Error bars represent s.e.m. Figure 6: Mitochondrial DNA levels and protein expression in the four lines of induced pluripotent stem cell (iPSC)-derived neurons. ( a–c ) Quantitative PCR measurement of three different segments of mitochondria DNA against the nuclear gene actin in the four lines of iPSC-derived neurons treated with or without CCCP (10 μM for 16 h). mtDNA3130-3301 is a region not transcribed and has no homology with mitochondrial pseudogenes in the nuclear genome. ( d ) Protein expression levels of PINK1 and DJ-1 in the absence or presence of CCCP treatment (10 μM for 24 h). PINK1 has two bands, uncleaved at 63 kDa and cleaved at 52 KDa. ( e ) The expression level of α-synuclein in the four lines of iPSC-derived neurons. Error bars represent s.e.m. Full size image One of the critical challenges for PD research is the lack of live human nigral DA neurons for mechanistic studies and drug discovery, as animal models of PD generally do not recapitulate the human condition very well [25] . The discovery of human iPSCs [8] , [9] makes it possible to generate patient-specific midbrain DA neurons to study their unique vulnerabilities in PD, particularly in monogenic forms of PD, in which the mechanistic link between genotype and phenotype is being vigorously pursued. The present study showed that parkin mutations directly impinge on dopamine utilization in human midbrain DA neurons. The loss of parkin significantly increased the spontaneous DA release that was independent of extracellular [Ca 2+ ] ( Fig. 4a ), but did not significantly affect Ca 2+ -dependent DA release triggered by membrane depolarization ( Fig. 4b ). It suggests that parkin limits somatodendritic DA release, which can be independent of extracellular [Ca 2+ ] [26] , [27] . As parkin is involved in vesicle trafficking through monoubiquitination of proteins such as Eps15 [28] , it seems plausible that parkin may affect the recycling of dopamine-containing vesicles that are involved in somatodendritic release. There is a strong feedback mechanism on the activity of TH, the rate-limiting enzyme in the synthesis of dopamine. It serves to maintain the homoeostasis of dopamine between cytosolic and vesicular pool so that increased release may be compensated by increased synthesis. In addition, VMAT2, DAT, MAO and COMT also impact on the homoeostasis of dopamine [29] . Thus, the total amount of endogenous dopamine was not significantly affected by parkin mutations ( Fig. 4d ). On the other hand, loss of parkin significantly decreased dopamine uptake ( Fig. 4f ) by reducing the total amount of correctly folded DAT ( Fig. 4h ). This is consistent with our previous finding that parkin increases the cell surface expression of DAT by ubiquitinating and degrading misfolded DAT conformers to enhance oligomerization of native DAT conformers in the endoplasmic reticulum and their subsequent delivery to the plasma membrane [18] . Recent positron emission tomography studies have shown that 18 F-DOPA uptake is significantly reduced in PD patients with parkin mutations, compared with controls [30] , [31] . Thus, mutations of parkin significantly disrupt the spatial and temporal precision of DA neurotransmission by increasing spontaneous DA release and decreasing DA uptake. The net outcome is increased extracellular DA level, which was mimicked by the dopamine treatment experiment in Figure 5a . In this paradigm, parkin mutations greatly increased dopamine-induced oxidative stress ( Fig. 5a,b ) because mutant parkin lost the ability to suppress MAO transcription ( Fig. 5c ). This result is consistent with our previous finding that parkin suppresses the transcription of monoamine oxidase A and B [17] . It appears that P002 had a particularly high level of MAO-B transcript ( Fig. 5c ) and activity ( Fig. 5d ), even when compared with P001. This might be related to different genetic background of the two patients and/or different parkin mutations that they carry (P002 has homozygous exon 3 deletion, while P001 has compound heterozygous deletion of exon 3 and exon 5). Overexpression of parkin, but not its PD-linked T240R mutant or GFP, rescued all the phenotypes—increased spontaneous DA release, decreased DA uptake and DAT-binding sites, increased MAO transcription and DA-induced oxidative stress ( Figs 4 and 5 ). Thus, these dopamine-specific phenotypes are indeed caused by loss-of-function mutations of parkin. Our findings on dopamine-specific functions of parkin also shed light on novel therapeutic targets of PD. Recent studies have shown that MAO-B inhibitors have a significant, albeit modest, effort in slowing down the progression of PD [32] . As parkin suppresses MAO transcription by ubiquitinating and degrading estrogen-related receptors [33] , it may be more advantageous to mimic the protective function of parkin by suppressing MAO transcription using inhibitors of estrogen-related receptors (for example, XCT-790) [34] , rather than inactivating MAO activity indiscriminately with suicide substrates such as those used in the current therapy. Alternatively, the ability of parkin to repress p53 [35] could also be exploited to achieve similar effects. On the other hand, agents that could enhance the folding of native DAT conformers or the elimination of misfolded DAT conformers may be good candidates to substitute parkin in restoring dopamine uptake. Agents that directly enhance DA uptake or increase the cell surface expression of DAT may also be suitable drug candidates. In conclusion, the study has discovered how mutations of parkin disrupt an essential function of human midbrain DA neurons—the coordinated utilization of dopamine as a neurotransmitter and the control of dopamine toxicity. Mechanistic insights gained from the study would be very useful for the development of disease-modifying therapies of PD on a platform that closely resembles human nigral DA neurons in vivo . Further studies are needed to address why nigral DA neurons, in comparison with other types of DA neurons, are particularly vulnerable in PD and how parkin protects against these vulnerabilities. Derivation of iPSCs from skin fibroblasts With approvals from the Health Sciences Institutional Review Board of the State University of New York at Buffalo and the Ethics Committee of Tottori University Faculty of Medicine, we obtained informed consents from research subjects participating in this study. Skin punch biopsies (5 mm in diameter or less) were obtained from two PD patients with parkin mutations and two control subjects. Skin fibroblasts (1×10 5 ) at passage 2 or 3 were infected for 16 h with the following FUW-tetO-LoxP lentiviruses: hOct4, hSox4, hKlf4 and hNanog each at MOI 15, c-Myc at MOI 6 and M2rtTA at MOI 30 in the presence of 4 μg ml −1 polybrene [10] . Doxycycline (1 μg ml −1 ) was added for at least 10 days and later at 0.5 μg ml −1 until hESC-like clones appeared. VPA (0.5 or 1 mM) was added for 7 days with DOX in the beginning. Clones with hESC morphology appeared between day 24 and 40. They were picked and expanded under hESC culture condition. The proviruses integrated in the genomes of the four iPSC lines were not removed because a recent study has demonstrated that neural differentiation of various iPSCs is not affected by the absence or presence of proviruses introduced during reprogramming [36] . Characterization of iPSCs The iPS cells were stained with SSEA-3 (1:1000, Millipore), SSEA-4 (1:1000, Millipore), TRA-1-60 (1:1000, Millipore), TRA-1-81 (1:1000, Millipore), Oct4 (1:1000, Millipore) and Nanog (1:500, Millipore). Alkaline phosphatase activity was detected using an alkaline phosphatase detection kit (Millipore). To confirm parkin mutations in iPS cells, RT–PCR was performed on total RNA isolated from iPSCs grown on matrigel. The complementary DNA region spanning exons 2–6 was amplified using two primers 5′-CACCTACCCAGTGACCATGATA-3′ and 5′-GCTACTGGTGTTTCCTTGTCAGA-3′. The PCR products were sequenced. DNA methylation states of the promoters of endogenous Oct4, Sox2 and Nanog were analysed using the Sequenom MassARRAY EpiTyper at Roswell Park Cancer Institute (PRCI) Genomics Shared Resource. Karyotyping of iPSCs grown on matrigel was performed by RPCI Sky Core Facility using Giemsa staining of iPSCs mitotically arrested at metaphase with colcimid. Chromosomes from at least 30 metaphase cells were analysed. Array comparative genomic hybridization of iPSCs was performed by the RPCI Genomics Shared Resource using commercially available, sex-mismatched pooled genomic DNA. The data have been deposited in GEO database under accession code GSE35190 . One million iPSCs mixed with collagen at a 1:1 ratio were aliquoted to ~10-μl pellets, which were grafted under the renal capsule of each kidney in a SCID mouse ( C.B-Igh-1bIcrTac-Prkdcscid/Ros ). Large tumours (~1 cm in size) were found for each iPSC line 2–3 months after grafting. All animal work for the teratoma formation assay was performed by RPCI Mouse Tumor Model Resource following RPCI IACUC-approved protocol. Directed differentiation of iPSCs to midbrain DA neurons The iPSCs were differentiated to midbrain DA neurons in a directed differentiation protocol [37] with two improvements. First, SB431542 (10 μM) was used for the first 4 days of iPSC-floating aggregates culture to enhance neural differentiation [12] . Second, matrigel was used in addition to polyornithine and laminin to coat the cell culture surface at the last step of differentiation (from neurosphere to neurons). Mature midbrain DA neurons capable of specific dopamine uptake were generated around day 70 from the start of differentiation. Dopamine release The iPSC-derived neuronal cultures differentiated at the same conditions in 6-well plates were treated at 37°C in the following way for each set of three wells (a, b and c). Well (a) was incubated in 1 ml HBSS for 30 min. Well (b) was incubated in 1 ml HBSS for 15 min and then 56 mM KCl was added for another 15 min. Well (c) was incubated in 1 ml HBSS without Ca 2+ and without Mg 2+ , but with 2 mM EDTA for 15 min and then 56 mM KCl was added for another 15 min. The 1-ml HBSS solutions were taken out from the wells. glutathione and EGTA were added to the solutions to the final concentration of 2 mM to prevent auto-oxidation of dopamine. The amounts of DA in HBSS solutions were measured by reverse phase HPLC (ESA Model 582 with ESA MD150×3.2 column, at 0.6 ml min −1 flow rate in MD-TM mobile phase) coupled with electrochemical detection [17] (ESA Coulochem III, E1: −250 mV, 2 μA; E2: 350 mV, 2 μA). Cells in the three wells were lysed in 0.5 N NaOH to measure protein levels, which were used to normalize dopamine release. Spontaneous dopamine release is reflected in (a), while Ca 2+ - and activity-dependent release is reflected in (b)–(c). Specific dopamine uptake The iPSC-derived neuronal cultures in 6-well plates were rinsed with 1 ml prewarmed uptake buffer (10 mM HEPES, 130 mM NaCl, 1.3 mM KCl, 2.2 mM CaCl 2 , 1.2 mM MgSO 4 , 1.2 mM KH 2 PO 4 , 10 mM glucose, pH 7.4) three times. Cells were incubated for 10 min at 37°C with 1 ml uptake buffer containing 5 μM dopamine without or with 10 μM nomifensine (a selective inhibitor of DAT). After the cells were washed at least three times in uptake buffer, they were lysed in 0.1 M perchloric acid with 1 mM EDTA and 0.1 mM sodium bisulphite. Cleared cell lysates were analysed for dopamine on HPLC coupled with electrochemical detection [17] (E1: −150 mV, 2 μA; E2: 220 mV, 2 μA). The pellets of cellular proteins were dissolved in 1 ml 0.5 N NaOH to measure protein contents, which were used to normalize dopamine uptake. Specific dopamine uptake is reflected in the difference of DA content in the absence and presence of the DAT inhibitor nomifensine. The amount of dopamine in the iPSC-derived neuronal cultures without any treatment was also measured. [ 3 H]CFT binding assay DAT radioligand binding assay using [ 3 H]CFT was performed with a protocol similar to what was described before [18] . After iPSC-derived neuronal cultures in 6-well plates were washed three times at room temperature in binding buffer (10 mM phosphate buffer, pH 7.4, 0.32 M sucrose), they were incubated in 1 ml of binding buffer containing 4 nM [ 3 H]CFT without or with the selective DAT inhibitor GBR12909 (10 μM) for 2 h at 4°C. The assay was terminated by three washes with 1 ml of ice-cold binding buffer. The neuronal cultures were lysed in 0.5 ml of 1% SDS for 15 min at room temperature and the entire lysate was measured in a scintillation counter. Non-specific binding was defined as binding in the presence of 10 μM GBR12909. It was subtracted from the total binding to derive specific [ 3 H]CFT binding. The total amounts of cellular proteins were measured in parallel experiments and used to normalize specific [ 3 H]CFT binding. Measurement of protein carbonyls The levels of protein carbonyls were measured as described before [38] . Protein carbonyls in total cell lysates containing 80 μg proteins were measured with the Oxyblot protein oxidation detection kit (Chemicon, Temecula, CA). Intensities of 2,4-dinitrophenyl (DNP)-modified proteins were quantified by densitometry. Background-subtracted signals were normalized against untreated C001 neural cultures. Electrophysiology Recordings of synaptic and ionic currents used standard whole-cell voltage-clamp techniques [39] . For the recording of spontaneous excitatory postsynaptic current, membrane potential was held at −70 mV. The external solution contained (mM): 127 NaCl, 5 KCl, 2 MgCl 2 , 2 CaCl 2 , 12 glucose and 10 HEPES, pH 7.3–7.4, 300–305 mOsm l −1 . To isolate AMPAR-mediated response, the NMDA receptor antagonist D -aminophosphonovalerate (20 μM) and GABA A receptor antagonist bicuculline (10 μM) were added. The internal solution consisted of the following (in mM): 130 Cs methanesulphonate, 10 CsCl, 4 NaCl, 10 HEPES, 1 MgCl 2 , 5 EGTA, 2.2 QX-314, 12 phosphocreatine, 5 MgATP, 0.5 Na 2 GTP and 0.1 leupeptin, pH 7.2–7.3, 265–270 mOsm. For the recording of NMDA-gated and GABA-gated currents, membrane potential was held at −60 mV or −40 mV, respectively. The internal solution contained the following (in mM): 180 N -methyl- D -glucamine, 40 HEPES, 4 MgCl 2 , 0.1 BAPTA, 12 phosphocreatine, 3 Na 2 ATP, 0.5 Na 2 GTP and 0.1 leupeptin, pH 7.2–7.3, 265–270 mOsm. The external solution consisted of the following (in mM): 127 NaCl, 20 CsCl, 10 HEPES, 1 CaCl 2 , 5 BaCl 2 , 12 glucose, 0.001 TTX and 0.02 glycine, pH 7.3–7.4, 300–305 mOsm. NMDA (100 μM) or GABA (100 μM) was applied to the cell for 2 s every 30 s to minimize desensitization-induced decrease of current amplitude. For the recording of APs, whole-cell current-clamp recordings were performed with the internal solution containing (in mM): 125 K-gluconate, 10 KCl, 10 HEPES, 0.5 EGTA, 3 Na 2 ATP, 0.5 Na 2 GTP and 12 phosphocreatine, pH 7.25, 280 mOsm. Cells were perfused with ACSF, and membrane potentials were kept at −55 to −65 mV. A series of hyperpolarizing and depolarizing step currents were injected to measure intrinsic properties and to elicit APs. Spontaneous APs were recorded without current injection. For the recording of voltage-dependent sodium and potassium currents, cells (held at −70mV) were perfused with ACSF, and voltage steps ranging from −90 mV to +50 mV were delivered at 10-mV increments. Data analyses were performed with Clampfit (Axon instruments) and Kaleidagraph (Albeck Software). Statistical analyses All statistical analyses were done with the software Origin (OriginLab, Northampton, MA). The data were expressed as mean±s.e.m. (standard error of measurement). Unpaired, two-tailed Student's t -tests were performed to evaluate whether the two groups were significantly different from each other. Accession codes: The aCGH data have been deposited in GEO database under accession code GSE35190 . How to cite this article: Jiang, H. et al . Parkin controls dopamine utilization in human midbrain dopaminergic neurons derived from induced pluripotent stem cells. Nat. Commun. 3:668 doi: 10.1038/ncomms1669 (2012).